Lysophosphatidylserine induces necrosis in pressure overloaded male mouse hearts via G protein coupled receptor 34 Heart failure is a leading cause of mortality in developed countries. Cell death is a key player in the development of heart failure. Calcium-independent phospholipase A 2 β (iPLA 2 β) produces lipid mediators by catalyzing lipids and induces nuclear shrinkage in caspase-independent cell death. Here, we show that lysophosphatidylserine generated by iPLA 2 β induces necrotic cardiomyocyte death, as well as contractile dysfunction mediated through its receptor, G protein-coupled receptor 34 (GPR34). Cardiomyocyte-specific iPLA 2 β-deficient male mice were subjected to pressure overload. While control mice showed left ventricular systolic dysfunction with necrotic cardiomyocyte death, iPLA 2 β-deficient mice preserved cardiac function. Lipidomic analysis revealed a reduction of 18:0 lysophosphatidylserine in iPLA 2 β-deficient hearts. Knockdown of Gpr34 attenuated 18:0 lysophosphatidylserine-induced necrosis in neonatal male rat cardiomyocytes, while the ablation of Gpr34 in male mice reduced the development of pressure overload-induced cardiac remodeling. Thus, the iPLA 2 β—lysophosphatidylserine—GPR34—necrosis signaling axis plays a detrimental role in the heart in response to pressure overload. Left ventricular (LV) dysfunction caused by various heart diseases, such as idiopathic dilated cardiomyopathy, ischemic heart diseases, valvular diseases, and myocarditis, leads to heart failure, a major cause of mortality in developed countries [1] . The mortality of heart failure remains high, although it has gradually improved for decades owing to modern treatment for this disease based on evidence obtained from a large number of clinical trials. Furthermore, because heart failure morbidity is high among the elderly [2] , the growing numbers of heart failure patients, along with high rehospitalization rates, will pose major social issues in aging societies. Thus, the identification of therapeutic targets and the development of novel therapies for heart failure constitute urgent priorities. Because cell death is known to be involved in the development and progression of LV dysfunction [3] , the regulation of cell death may be one of the best options for a novel heart failure therapy. However, a therapy suppressing cell death has not yet been established as a heart failure treatment. Phospholipase A 2 (PLA 2 ) hydrolyzes the sn −2 bond in phospholipids to release free fatty acids and lysophospholipids [4] . The PLA 2 superfamily consists of several families, including secretory PLA 2 , cytosolic calcium-dependent PLA 2 , and calcium-independent phospholipase A 2 (iPLA 2 ) [5] . iPLA 2 s catalyze and maintain homeostasis or remodeling of membrane phospholipids and play a role in cellular signal transduction. Among iPLA 2 subtypes, iPLA 2 β is the most studied and best understood [6] . iPLA 2 β is localized in the cytosol under the basal condition; in stimulatory conditions, it is translocated to the mitochondria, ER, and nucleus [6] . Shinzawa et al. reported that iPLA 2 β is required for caspase-independent cell death characterized by nuclear shrinkage [7] . Thus, we hypothesized that iPLA 2 β and its product may be involved in the pathogenesis of LV dysfunction by inducing cell death. The aim of this study is to investigate the pathophysiological role of iPLA 2 β in the mouse heart. We found that iPLA 2 β plays a detrimental role in the development of pressure-overloaded cardiac dysfunction by inducing necrotic, but not apoptotic, cell death via G protein-coupled receptor (GPR) 34. Cardiomyocyte-specific calcium-independent phospholipase A 2 β-deficient mice showed no significant cardiac phenotypes under normal conditions To investigate the in vivo role of iPLA 2 β in the heart, we generated cardiomyocyte-specific iPLA 2 β-deficient mice. Floxed mice of Pla2g6 , encoding iPLA 2 β, were generated (Supplementary Fig. 1a, b ) and then crossed with transgenic mice expressing Cre recombinase under the control of the α-myosin heavy chain promoter ( Myh6 ) to obtain cardiomyocyte-specific iPLA 2 β-deficient mice: Pla2g6 flox/flox ; Myh6-Cre + mice ( Pla2g6 −/− ). The Pla2g6 flox/flox ; Myh6-Cre − littermates ( Pla2g6 +/+ ) were used as controls. Schematic structures of genomic Pla2g6 sequences and the targeting vector are shown in Supplementary Fig. 1a . Homogenous recombinants were identified by Southern blotting (Supplementary Fig. 1b ). The Pla2g6 −/− mice were born at the expected Mendelian frequency (male Pla2g6 +/+ : male Pla2g6 −/− : female Pla2g6 +/+ : female Pla2g6 −/− = 77:62:55:49) and were indistinguishable from their littermates. The mice grew to adulthood and showed normal fertility. Western blot analysis demonstrated that the cardiomyocyte-specific ablation of Pla2g6 gene resulted in a significant reduction of iPLA 2 β protein expression in cardiomyocytes isolated from the heart (Supplementary Fig. 1c ). The Pla2g6 ablation had no significant impact on the expression levels of iPLA 2 β in all tissues investigated except the heart (Supplementary Fig. 1d ). The levels of the other iPLA 2 subtypes were not changed in cardiomyocytes or non-cardiomyocytes isolated from the heart (Supplementary Fig. 1e, f ). The expression level of iPLA 2 β was not altered in Pla2g6 −/− non-cardiomyocytes (Supplementary Fig. 1f ). 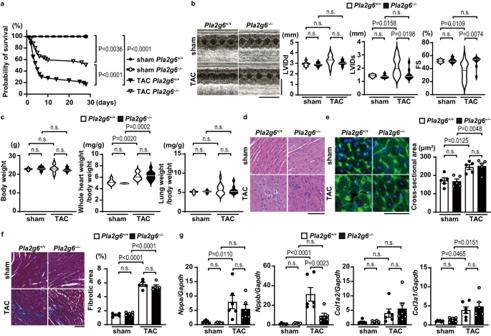Fig. 1: Cardiac phenotypes of cardiac-specific iPLA2β-deficient mice after pressure overload. ThePla2g6+/+andPla2g6–/–mice were subjected to transverse aortic constriction (TAC) and then analyzed 5 days after the operation.aSurvival ratio after TAC.n= 17 (sham-operatedPla2g6+/+), 13 (sham-operatedPla2g6–/–), 51 (TAC-operatedPla2g6+/+), and 51 (TAC-operatedPla2g6–/–). The log-rank test was used for survival analysis. ShamPla2g6+/+versus TACPla2g6+/+P= 0.0000001, TACPla2g6+/+versus TACPla2g6–/–P= 0.0002.bRepresentative images of transthoracic M-mode echocardiographic tracing (scale bars, 0.2 s and 5 mm, respectively) and the echocardiographic parameters of the mice.n= 7 (sham-operatedPla2g6+/+), 7 (sham-operatedPla2g6–/–), 14 (TAC-operatedPla2g6+/+) and 10 (TAC-operatedPla2g6–/–). LVIDd and LVIDs, end-diastolic and end-systolic left ventricular (LV) internal dimensions; FS, fractional shortening of LV.cPhysiological parameters of the mice.n= 7 (sham-operatedPla2g6+/+), 7 (sham-operatedPla2g6–/–), 14 (TAC-operatedPla2g6+/+), and 10 (TAC-operatedPla2g6–/–), biologically independent samples.dRepresentative images of the hematoxylin—eosin-stained heart sections. Experiment was repeated five times independently with similar results. Scale bar, 100 μm.eRepresentative images of the wheat germ agglutinin (green)-stained heart sections. Scale bar, 50 μm. Blue, DAPI. The graph shows the cross-sectional area of cardiomyocytes (n= 5, biologically independent samples).fRepresentative images of Azan—Mallory-stained heart sections. Scale bar, 100 μm. The graph shows the ratio of the fibrotic area to whole heart section (n= 5, biologically independent samples. ShamPla2g6+/+versus TACPla2g6+/+P= 0.0000000002, shamPla2g6–/–versus TACPla2g6–/–P= 0.000000001).gExpression levels of mRNAs related to cardiac remodeling. (n= 6, biologically independent samples. ShamPla2g6+/+versus TACPla2g6+/+inNppb/Gapdh P= 0.00006). Data were normalized to theGapdhcontent and are expressed as the fold increase over the levels in the sham-operatedPla2g6+/+group. Open and closed bars indicatePla2g6+/+andPla2g6−/−, respectively. In violin plots, solid lines show median. In bar graphs, data are expressed as the mean ± SEM. The data were evaluated by one-way ANOVA, followed by Tukey-Kramer’spost-hoctest. Source data are provided as a Source Data file. 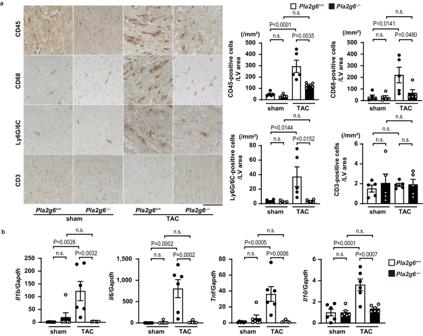Fig. 2: Inflammatory responses in TAC-operatedPla2g6−/−hearts. ThePla2g6+/+andPla2g6–/–mice were subjected to transverse aortic constriction (TAC) and then analyzed 5 days after the operation.aRepresentative images of immunohistochemical analysis of CD45, CD68, Ly6G/6C and CD3. Scale bar, 100 μm. The graphs show quantitative analysis of each infiltrating inflammatory cell type (n= 5, biologically independent samples. ShamPla2g6+/+versus TACPla2g6+/+in CD45-positive cells/LV areaP= 0.00007). LV area, left ventricular area.bExpression levels of mRNAs related to inflammatory responses. The levels of mRNA were analyzed 5 days after the operation (n= 6, biologically independent samples). Data were normalized to theGapdhcontent and are expressed as the fold increase over the levels in the sham-operatedPla2g6+/+group. Open and closed bars indicatePla2g6+/+andPla2g6−/−, respectively. Data are expressed as the mean ± SEM. The data were evaluated by one-way ANOVA, followed by Tukey-Kramer’spost-hoctest. Source data are provided as a Source Data file. No significant differences between Pla2g6 −/− and Pla2g6 +/+ mice were observed in any echocardiographic (Supplementary Table 1 ) or physiological (Supplementary Table 2 ) parameters at 10 weeks of age. Cardiomyocyte-specific ablation of Pla2g6 attenuated the development of cardiac dysfunction in response to pressure overload Pla2g6 +/+ and Pla2g6 −/− mice were subjected to pressure overload by means of transverse aortic constriction (TAC) surgery, in order to examine the in vivo role of iPLA 2 β during cardiac remodeling. Twenty-eight days after TAC, 82.7% of Pla2g6 +/+ mice had died, whereas 51.9% of Pla2g6 −/− mice were still alive (Fig. 1a ). To analyze the phenotypes observed in Pla2g6 −/− mice, the mouse hearts were evaluated 5 days after TAC operation when half of the TAC-operated Pla2g6 +/+ mice remained alive. On day 5 after TAC operation, echocardiographic analysis showed that end-systolic LV internal dimension (LVIDs) in the Pla2g6 +/+ hearts were larger and fractional shortening of LV (FS) was lower than sham-operated controls. End-diastolic LV internal dimension (LVIDd) showed no significant difference between the two groups. Those indicate LV systolic dysfunction without LV dilatation in the TAC-operated Pla2g6 +/+ hearts. The ablation of Pla2g6 attenuated the changes in LVIDs and FS after TAC (Fig. 1b ). Although there was no significant difference in body weight, the whole heart-to-body weight ratio, an index for cardiac hypertrophy, was increased in both TAC groups to a similar extent compared to that observed in the corresponding controls (Fig. 1c ). There was no significant increase in the lung-to-body weight ratio, an index for lung congestion. Histological analyses show cellular infiltration (Fig. 1d ) and an increase in the cardiomyocyte cross-sectional area, a marker for cardiac hypertrophy (Fig. 1e ), as well as an increased fibrotic area (Fig. 1f ) in both TAC-operated groups; however, there were no significant differences between the two groups. The mRNA expression levels of Nppa , a marker for cardiac hypertrophy, and Col1a2 and Col3a1 , markers for fibrosis, did not show significant differences between the TAC-operated Pla2g6 +/+ and Pla2g6 −/− groups (Fig. 1g ). The level of Nppb mRNA, a marker for cardiac remodeling, in the TAC-operated Pla2g6 +/+ group was higher than that in the TAC-operated Pla2g6 −/− group (Fig. 1g ). Fig. 1: Cardiac phenotypes of cardiac-specific iPLA 2 β-deficient mice after pressure overload. The Pla2g6 +/+ and Pla2g6 –/– mice were subjected to transverse aortic constriction (TAC) and then analyzed 5 days after the operation. a Survival ratio after TAC. n = 17 (sham-operated Pla2g6 +/+ ), 13 (sham-operated Pla2g6 –/– ), 51 (TAC-operated Pla2g6 +/+ ), and 51 (TAC-operated Pla2g6 –/– ). The log-rank test was used for survival analysis. Sham Pla2g6 +/+ versus TAC Pla2g6 +/+ P = 0.0000001, TAC Pla2g6 +/+ versus TAC Pla2g6 –/– P = 0.0002. b Representative images of transthoracic M-mode echocardiographic tracing (scale bars, 0.2 s and 5 mm, respectively) and the echocardiographic parameters of the mice. n = 7 (sham-operated Pla2g6 +/+ ), 7 (sham-operated Pla2g6 –/– ), 14 (TAC-operated Pla2g6 +/+ ) and 10 (TAC-operated Pla2g6 –/– ). LVIDd and LVIDs, end-diastolic and end-systolic left ventricular (LV) internal dimensions; FS, fractional shortening of LV. c Physiological parameters of the mice. n = 7 (sham-operated Pla2g6 +/+ ), 7 (sham-operated Pla2g6 –/– ), 14 (TAC-operated Pla2g6 +/+ ), and 10 (TAC-operated Pla2g6 –/– ), biologically independent samples. d Representative images of the hematoxylin—eosin-stained heart sections. Experiment was repeated five times independently with similar results. Scale bar, 100 μm. e Representative images of the wheat germ agglutinin (green)-stained heart sections. Scale bar, 50 μm. Blue, DAPI. The graph shows the cross-sectional area of cardiomyocytes ( n = 5, biologically independent samples). f Representative images of Azan—Mallory-stained heart sections. Scale bar, 100 μm. The graph shows the ratio of the fibrotic area to whole heart section ( n = 5, biologically independent samples. Sham Pla2g6 +/+ versus TAC Pla2g6 +/+ P = 0.0000000002, sham Pla2g6 –/– versus TAC Pla2g6 –/– P = 0.000000001). g Expression levels of mRNAs related to cardiac remodeling. ( n = 6, biologically independent samples. Sham Pla2g6 +/+ versus TAC Pla2g6 +/+ in Nppb/Gapdh P = 0.00006). Data were normalized to the Gapdh content and are expressed as the fold increase over the levels in the sham-operated Pla2g6 +/+ group. Open and closed bars indicate Pla2g6 +/+ and Pla2g6 −/− , respectively. In violin plots, solid lines show median. In bar graphs, data are expressed as the mean ± SEM. The data were evaluated by one-way ANOVA, followed by Tukey - Kramer’s post-hoc test. Source data are provided as a Source Data file. Full size image Moon et al. reported that iPLA 2 γ in the myocardium is activated and plays a detrimental role in the response to ischemic reperfusion injury [8] . The protein expression level of iPLA 2 γ was not increased after TAC operation in wild-type C57BL/6J mouse hearts, while that of iPLA 2 β was significantly increased with a peak at 3 days after TAC (Supplementary Fig. 2a ). In addition, there were no significant differences in the protein expression levels of iPLA 2 γ in sham or TAC-operated Pla2g6 +/+ and Pla2g6 −/− hearts 3 days after operation (Supplementary Fig. 2b ). Inflammatory responses were downregulated in Pla2g6 −/− hearts after TAC Next, inflammatory responses in the heart after TAC were evaluated using immunohistochemical analysis (Fig. 2a ). Five days after the operation, TAC-operated Pla2g6 +/+ hearts showed significant increases in the infiltration of CD45 + cells, including CD68 + macrophages and Ly6G/6C + neutrophils, but not CD3 + lymphocytes in the mouse LV. The mRNA levels of interleukin (IL)−1β ( Il1b ), IL-6 ( Il6 ), tumor necrosis factor (TNF)-α ( Tnf ), and IL-10 ( Il10 ) were significantly upregulated in TAC-operated Pla2g6 +/+ mouse hearts. The ablation of Pla2g6 attenuated these TAC-induced inflammatory responses (Fig. 2a, b ). Fig. 2: Inflammatory responses in TAC-operated Pla2g6 −/− hearts. The Pla2g6 +/+ and Pla2g6 –/– mice were subjected to transverse aortic constriction (TAC) and then analyzed 5 days after the operation. a Representative images of immunohistochemical analysis of CD45, CD68, Ly6G/6C and CD3. Scale bar, 100 μm. The graphs show quantitative analysis of each infiltrating inflammatory cell type ( n = 5, biologically independent samples. Sham Pla2g6 +/+ versus TAC Pla2g6 +/+ in CD45-positive cells/LV area P = 0.00007). LV area, left ventricular area. b Expression levels of mRNAs related to inflammatory responses. The levels of mRNA were analyzed 5 days after the operation ( n = 6, biologically independent samples). Data were normalized to the Gapdh content and are expressed as the fold increase over the levels in the sham-operated Pla2g6 +/+ group. Open and closed bars indicate Pla2g6 +/+ and Pla2g6 −/− , respectively. Data are expressed as the mean ± SEM. The data were evaluated by one-way ANOVA, followed by Tukey - Kramer’s post-hoc test. Source data are provided as a Source Data file. Full size image Necrotic, but not apoptotic, cell death was inhibited in TAC-operated Pla2g6 −/− hearts To investigate the mechanism underlying the phenotypes observed in the Pla2g6 −/− mice, the effect of iPLA 2 β deficiency on cell death was examined in TAC-operated mouse hearts. First, TUNEL (terminal deoxynucleotidyl transferase-mediated dUTP-biotin nick-end labeling) staining was performed to evaluate apoptosis. Although both TAC-operated groups showed an elevated number of apoptotic cardiomyocytes, there was no difference between the two groups (Fig. 3a ). Next, we investigated necrotic cell death, which is characterized by the leakage of cellular components, hyperpermeability in the cell membrane, and the release of damage-associated molecular patterns (DAMPs) [9] . To evaluate the leakage of cardiomyocyte cellular components into circulation, serum troponin T concentrations were measured. The ablation of Pla2g6 attenuated the elevation of serum troponin T concentration after TAC operation (Fig. 3b ). Then, membrane permeability was tested by examining the uptake of Evans blue dye into the hearts. The sporadic Evans blue dye-positive area was larger in TAC-operated Pla2g6 +/+ hearts than in TAC-operated Pla2g6 −/− or corresponding sham-operated hearts (Fig. 3c ). Because high mobility group box 1 (HMGB1) is a well-known DAMP [10] , we examined the release of HMGB1 from nuclei in cardiomyocytes after TAC. A significant increase in the number of nuclei that lost the signal of HMGB1 was observed in Pla2g6 +/+ hearts. However, this number was significantly smaller in Pla2g6 −/− hearts than in Pla2g6 +/+ hearts (Fig. 3d ). Fig. 3: Decrease in necrotic cell death in TAC-operated Pla2g6 −/− hearts. The Pla2g6 +/+ and Pla2g6 –/– mice were subjected to transverse aortic constriction (TAC) and then analyzed 5 days after the operation. a Representative confocal images of TUNEL-positive cardiomyocytes. Arrow heads indicate TUNEL (green)-positive nuclei. Scale bar, 20 μm. Red, α-sarcomeric actin; blue, DAPI. The graph shows quantitative analysis of TUNEL-positive cardiomyocytes ( n = 5, biologically independent samples). b Serum troponin T levels. n = 5 (sham-operated Pla2g6 +/+ ), 5 (sham-operated Pla2g6 –/– ), 8 (TAC-operated Pla2g6 +/+ ), and 8 (TAC-operated Pla2g6 –/– ), biologically independent samples. c Uptake of Evans blue dye (red) in the hearts of Pla2g6 +/+ and Pla2g6 –/– mice following TAC or sham operation. Scale bar, 1 mm. The graph shows the ratio of Evans blue dye-positive area to left ventricular area. n = 5 (sham-operated Pla2g6 +/+ ), 5 (sham-operated Pla2g6 –/– ), 7 (TAC-operated Pla2g6 +/+ ), and 7 (TAC-operated Pla2g6 –/– ) biologically independent samples. d Immunofluorescence analysis of HMGB1 (green) and α-sarcomeric actin (red) in the heart after TAC ( n = 5, biologically independent samples. Sham Pla2g6 +/+ versus TAC Pla2g6 +/+ P = 0.00002). Arrow heads indicate HMGB1-negative nuclei. Scale bar, 50 μm. Blue, DAPI. The graph shows the percentage of HMGB1-negative cardiomyocytes. Open and closed bars indicate Pla2g6 +/+ and Pla2g6 −/− , respectively. Data are expressed as the mean ± SEM. The data were evaluated by one-way ANOVA, followed by Tukey-Kramer’s post - hoc test. Source data are provided as a Source Data file. Full size image Lysophosphatidylserine was increased under pressure overload in the heart We hypothesized that free fatty acid or lysophospholipid produced by iPLA 2 β in cardiomyocytes was responsible for the differences in the cardiac phenotypes observed in Pla2g6 +/+ and Pla2g6 −/− hearts under pressure overload. To verify this hypothesis, we performed untargeted lipidomic analysis in heart tissues. We hypothesized that the level of a candidate lipid would be increased in TAC-operated Pla2g6 +/+ hearts in response to pressure overload and that the ablation of Pla2g6 would attenuate this increase. Heat maps showed the contents of 298 molecular species of lipids detected in TAC-operated hearts (Fig. 4a , Supplementary Fig. 3 ). The amount of 10 lipids in the TAC-operated Pla2g6 +/+ group was significantly higher than that in the sham-operated Pla2g6 +/+ group or the TAC-operated Pla2g6 −/− group (Fig. 4b and Supplementary Fig. 4 ). Among them, only 18:0 lysophosphatidylserine can be a product derived from hydrolysis by iPLA 2 β, suggesting that 18:0 lysophosphatidylserine is involved in pressure overload-induced cardiac remodeling. Fig. 4: Untargeted lipidomic analysis of free fatty acids and lysophospholipids released in TAC-operated Pla2g6 −/− heart tissue. a Heat map showing the contents of molecular species of free fatty acids and lysophospholipids in mouse hearts after TAC operation. Correlation of peak values and color is indicated at the top; High, red and low, blue. Red arrow indicates 18:0 lysophosphatidylserine. LPS lysophosphatidylserine, LPI lysophosphatidylinositol, LPG lysophosphatidylglucoside, LPE lysophosphatidylethanolamine, LPC lysophosphatidylcholine, FA free fatty acid. b Quantity of 18:0 lysophosphatidylserine in mouse hearts after TAC operation. n = 4 (sham-operated Pla2g6 +/+ ), 4 (sham-operated Pla2g6 –/– ), 5 (TAC-operated Pla2g6 +/+ ), and 5 (TAC-operated Pla2g6 –/– ), biologically independent samples. Average values of each group were used for heat map analysis ( a ). Open and closed bars indicate Pla2g6 +/+ and Pla2g6 −/− , respectively ( b ). Data are expressed as the mean ± SEM. The data were evaluated by one-way ANOVA, followed by Tukey-Kramer’s post-hoc test. Source data are provided as a Source Data file. Full size image It has been reported that ischemia-activated iPLA 2 s degrade plasmalogens in myocardium [11] . The lipidomic analysis revealed that no plasmalogens showed significant iPLA 2 β-dependent changes in the response to pressure-overload, except 18:1/18:2 plasmalogen (Supplementary Fig. 5a ). Free fatty acids are produced following the degradation of plasmalogen by phospholipase A 2 [12] . However, our data indicate no significant increase in the amount of 18:1 or 18:2 free fatty acid after TAC (Supplementary Fig. 5b ). Moon et al. has reported several possible lipid mediators involved in the iPLA 2 γ-mediated cardiac injury [8] . Our data showed the mediators were not significantly increased in Pla2g6 +/+ or Pla2g6 −/− hearts after TAC (Supplementary Fig. 6 ). 18:0 lysophosphatidylserine induced necrotic cell death via G protein-coupled receptor 34 in rat neonatal cardiomyocytes To elucidate the role of 18:0 lysophosphatidylserine in inducing cell death and heart failure, we investigated the association between lysophosphatidylserine and cell death using isolated primary rat neonatal cardiomyocytes. The cell viability assay reveals that lysophosphatidylserine induced cell death in rat neonatal cardiomyocytes in both time- and dose-dependent manners (Fig. 5a, b ). Live, necrotic, early apoptotic and late apoptotic cells were identified as PI (propidium iodide) − TUNEL − , PI + TUNEL − , PI − TUNEL + and PI + TUNEL + cells, respectively. Immunocytochemical analysis shows that necrotic cell death was induced by treatment with lysophosphatidylserine in cardiomyocytes (Fig. 5c ). Fig. 5: 18:0 lysophosphatidylserine-induced cell death in rat neonatal cardiomyocytes. a , b Cell viability assay. Cell viability was measured using the Cell Titer-Blue Assay Kit. Isolated rat neonatal cardiomyocytes were treated with 50 μM 18:0 lysophosphatidylserine for the indicated time, or with the indicated concentration of 18:0 lysophosphatidylserine for 12 h. The percentage of cell viability is shown in the graphs ( n = 5). The data were evaluated by one-way ANOVA, followed by Tukey-Kramer’s post - hoc test. c Immunofluorescent analysis of TUNEL (green), propidium iodide (PI) (red) and DAPI (blue) stained-neonatal cardiomyocytes after stimulation with 50 μM 18:0 lysophosphatidylserine (LPS) for 12 h. Scale bars, 50 μm. Necrosis was assessed by PI + and TUNEL – , while early apoptosis was assessed by PI – and TUNEL + and late apoptosis was assessed by PI + and TUNEL + . The bottom graphs show quantitative analysis ( n = 5). Two-sided unpaired Student’s t- test was used for analysis (EtOH versus LPS in Percentage of PI – TUNEL – cells P = 0.00006). 1% (v/v) ethanol (EtOH) was used as the control sample. d , e The effect of knockdown of LPS receptors on cell viability. Isolated neonatal cardiomyocytes were transfected with siRNAs targeting GPR34 or GPR132 (siGPR34 or siGPR132) or with negative control siRNA (siNC). These cells were treated with 50 μM LPS for 12 h. The percentage of cell viability is shown in the graphs ( n = 12). The data were analyzed by one-way ANOVA, followed by Tukey-Kramer’s post-hoc test (siNC EtOH versus siNC LPS in ( d , e ) P = 0.0000005 and P = 0.0000007, respectively, siGPR132 EtOH versus siGPR132 LPS P = 0.000002). Open and closed bars indicate siNC and siGPR34 or siGPR132, respectively. f Immunofluorescent analysis of TUNEL, PI and DAPI stained-cardiomyocytes after stimulation with 50 μM LPS for 12 h under the condition of GPR34 knockdown. Scale bar, 50 μm. The graphs show quantitative analysis ( n = 9). The data were evaluated by one-way ANOVA, followed by Tukey-Kramer’s post - hoc test. Open and closed bars indicate siNC and siGPR34, respectively. In violin plots, solid lines show median. In bar graphs, data are expressed as the mean ± SEM. Source data are provided as a Source Data file. Full size image Lysophosphatidylserine is also known to be a ligand for GPRs [13] , [14] , [15] , [16] , [17] . Although GPR34, GPR132, GPR174, and P2Y10 have been identified as the responsible receptors for lysophosphatidylserine, GPR174 and P2Y10 are known to be exclusively expressed in immune-related tissues and to have an inhibitory role in immune responses mainly [18] . We investigated the functions of these receptors in lysophosphatidylserine-stimulated cardiomyocyte death in primary isolated neonatal rat cardiomyocytes. The expression of GPR34 or GPR132 mRNA and protein was detected in cardiomyocytes in agreement with the previous reports [13] , [19] . The expressions were suppressed using small interfering RNA (siRNA) (Supplementary Fig. 7a, b ). Knockdown of GPR34 protein expression reduced lysophosphatidylserine-induced cell death, although knockdown of GPR132 did not (Fig. 5d, e ). In addition, immunocytochemical analysis indicates that GPR34 knockdown inhibited lysophosphatidylserine-induced PI + TUNEL − necrotic cell death (Fig. 5f ). Next, we attempted to obtain experimental evidence connecting lysophosphatidylserine with GPR34 in cardiomyocytes. It has been reported that lysophosphatidylserine decreased forskolin-induced cyclic adenosine monophosphate (cAMP) accumulation mediated through GPR34 [13] , [14] . In neonatal rat cardiomyocytes, lysophosphatidylserine stimulation decreased forskolin-induced cAMP accumulation in a dose-dependent manner (Supplementary Fig. 7c ), and knockdown of GPR34 attenuated the inhibitory effect of lysophosphatidylserine on the cAMP accumulation (Supplementary Fig. 7d ). To examine how lysophosphatidylserine-activated GPR34 signals to necrotic cardiomyocyte death, we evaluated protein expression levels of receptor interacting serine/threonine kinase 1 and 3 (RIP1 and RIP3) in rat neonatal cardiomyocytes treated with lysophosphatidylserine. Treatment with lysophosphatidylserine increased the protein expression levels of RIP3 and phospho-RIP3 in control cells, but not in GPR34-knockdown cells. It had no effect on those of RIP1 and phospho-RIP1 (Supplementary Fig. 7e ). Gpr34 ablation attenuated the development of cardiac dysfunction induced by pressure overload To examine the involvement of lysophosphatidylserine-dependent necrosis mediated by GPR34 in the pathogenesis of pressure overload-induced heart failure, control wild-type C57BL/6J mice ( Gpr34 +/+ ) and GPR34-deficient mice ( Gpr34 −/− ) were subjected to TAC and then analyzed 5 days after TAC. Gpr34 mRNA was expressed in cardiomyocytes isolated from adult Gpr34 +/+ hearts and completely deleted in Gpr34 −/− cardiomyocytes (Supplementary Fig. 8 ). 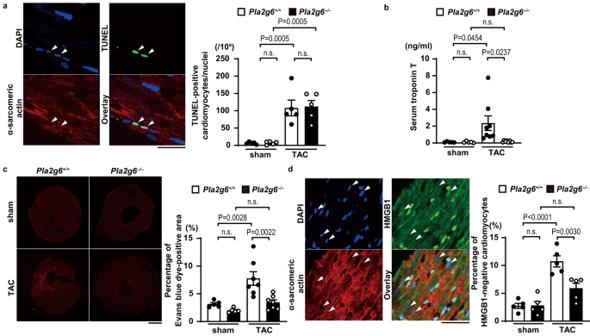Fig. 3: Decrease in necrotic cell death in TAC-operatedPla2g6−/−hearts. ThePla2g6+/+andPla2g6–/–mice were subjected to transverse aortic constriction (TAC) and then analyzed 5 days after the operation.aRepresentative confocal images of TUNEL-positive cardiomyocytes. Arrow heads indicate TUNEL (green)-positive nuclei. Scale bar, 20 μm. Red, α-sarcomeric actin; blue, DAPI. The graph shows quantitative analysis of TUNEL-positive cardiomyocytes (n= 5, biologically independent samples).bSerum troponin T levels.n= 5 (sham-operatedPla2g6+/+), 5 (sham-operatedPla2g6–/–), 8 (TAC-operatedPla2g6+/+), and 8 (TAC-operatedPla2g6–/–), biologically independent samples.cUptake of Evans blue dye (red) in the hearts ofPla2g6+/+andPla2g6–/–mice following TAC or sham operation. Scale bar, 1 mm. The graph shows the ratio of Evans blue dye-positive area to left ventricular area.n= 5 (sham-operatedPla2g6+/+), 5 (sham-operatedPla2g6–/–), 7 (TAC-operatedPla2g6+/+), and 7 (TAC-operatedPla2g6–/–) biologically independent samples.dImmunofluorescence analysis of HMGB1 (green) and α-sarcomeric actin (red) in the heart after TAC (n= 5, biologically independent samples. ShamPla2g6+/+versus TACPla2g6+/+P= 0.00002). Arrow heads indicate HMGB1-negative nuclei. Scale bar, 50 μm. Blue, DAPI. The graph shows the percentage of HMGB1-negative cardiomyocytes. Open and closed bars indicatePla2g6+/+andPla2g6−/−, respectively. Data are expressed as the mean ± SEM. The data were evaluated by one-way ANOVA, followed by Tukey-Kramer’spost-hoctest. Source data are provided as a Source Data file. There were no significant differences between Gpr34 +/+ and Gpr34 −/− mice in their echocardiographic parameters at baseline (Supplementary Table 3 ). Compared to sham-operated controls, pressure overload increased LVIDd and LVIDs and reduced FS in Gpr34 +/+ mice (Fig. 6a ). Gpr34 −/− mice showed reduced LV chamber dilation and cardiac dysfunction. TAC-operated Gpr34 +/+ mice showed an increase in cellular infiltration (Fig. 6b ) and necrotic cell death, as indicated by HMGB1 release from nuclei (Fig. 6c ). Both cellular infiltration and necrotic cell death were inhibited by the ablation of Gpr34 . On the other hand, the number of TUNEL-positive cardiomyocytes did not differ between the two TAC-operated groups (Fig. 6d ). Fig. 6: The protective effect of GPR34 deficiency from pressure overload in the heart. Gpr34 +/+ and Gpr34 –/– mice were subjected to TAC and then analyzed 5 days after the operation. a Representative images of transthoracic M-mode echocardiographic tracing. Scale bars, 0.2 s and 5 mm, respectively. The graphs show echocardiographic parameters of the mice ( n = 7, biologically independent samples. Sham Gpr34 +/+ versus TAC Gpr34 +/+ in LVIDs and FS P = 0.0000000001 and P = 0.0000002, respectively, TAC Gpr34 +/+ versus TAC Gpr34 –/– in LVIDs and FS P = 0.000000006 and P = 0.00006, respectively). b Representative images of the hematoxylin-eosin-stained heart sections. Experiment was repeated five times independently with similar results. Scale bar, 100 μm. c Immunofluorescence analysis of HMGB1 (green), α-sarcomeric actin (red) and DAPI (blue) in the heart after TAC ( n = 5, biologically independent samples. Sham Gpr34 +/+ versus TAC Gpr34 +/+ P = 0.000002). Arrow heads indicate HMGB1-negative nuclei. Scale bar, 50 μm. The graph shows the percentage of HMGB1-negative cardiomyocytes. d Representative confocal images of TUNEL (green)-positive cardiomyocytes. Arrow heads indicate TUNEL-positive nuclei. Scale bar, 50 μm. Red, α-sarcomeric actin; blue, DAPI. The graph shows quantitative analysis of TUNEL-positive cardiomyocytes. ( n = 7, biologically independent samples). Open and closed bars indicate Gpr34 +/+ and Gpr34 −/− , respectively. Data are expressed as the mean ± SEM. The data were evaluated by one-way ANOVA, followed by Tukey-Kramer’s post-hoc test. Source data are provided as a Source Data file. Full size image In this study, we attempt to elucidate the role of iPLA 2 β in cardiomyocyte death and cardiac remodeling. Pla2g6 −/− mice showed no cardiac phenotypes at baseline, indicating that there is no cardiomyocyte-autonomous requirement for iPLA 2 β during normal embryonic development or postnatal heart growth. iPLA 2 β deficiency attenuated cardiac dysfunction, but not cardiac hypertrophy induced by TAC. Thus, we posit that iPLA 2 β is detrimental to the heart in response to pressure overload. It has been reported that iPLA 2 β is activated during cardiac ischemia [20] and upregulated after reperfusion [21] , and that the inhibition and downregulation of iPLA 2 β reduce infarct size after ischemia reperfusion injury [21] , [22] . These studies align with our results regarding the detrimental role of iPLA 2 β in stressed hearts. However, iPLA 2 β-deficient mice showed neuroaxonal dystrophy with spheroids and vacuoles [4] , [23] , progressive motor disorders, and age-related neuropathology [24] , suggesting its protective role. Furthermore, even in the same tissues or cell types, the role of iPLA 2 β is contradictory [6] , [25] , [26] , [27] . The intracellular localization of iPLA 2 β changes dynamically depending on tissues and stimuli [7] , [28] , [29] , which may explain why the effects of iPLA 2 β appear to be a double-edged sword. It has been reported that cell death, including both apoptosis and necrosis, is involved in the development and progression of heart failure [3] . Our data suggest that iPLA 2 β in cardiomyocytes plays an important role in the induction of necrotic cell death but not apoptosis in response to pressure overload. Furthermore, the present study shows that the ablation of iPLA 2 β attenuated inflammatory responses in the heart after TAC. However, we cannot conclude whether necrosis or inflammation is a primary cause for this cardiac dysfunction. The membrane-associated iPLA 2 γ has been shown to be the predominant isoform activated with myocardial injury [8] . We showed pressure overload increased the level of iPLA 2 β protein in the heart, while it had no effect on that of iPLA 2 γ. In addition, our lipidomics data showed reported mediators involved in iPLA 2 γ-mediated cardiac injury were not significantly increased in Pla2g6 +/+ hearts after TAC [8] . These results suggest no potential contribution of iPLA 2 γ to pressure overload-induced cardiac remodeling. We performed untargeted lipidomic analysis to identify lipids responsible for the phenotypes observed in TAC-operated Pla2g6 −/− hearts. We hypothesized that pressure overload would lead to a Pla2g6 -dependent increase in the level of a candidate lipid. Although 10 lipids met the criteria, only 18:0 lysophosphatidylserine can be produced by iPLA 2 β. A very high abundance of plasmalogens in myocardial membrane has been reported and hydrolysis of plasmalogens is prominent in myocardial pathophysiology [11] , [30] . Our lipidomics data suggest that plasmalogens were not involved in the mechanism underlying the phenotypes observed in Pla2g6 −/− mice. Thus, 18:0 lysophosphatidylserine was likely to be a responsible candidate. Lysophosphatidylserine is produced through the diacylation of phosphatidylserine by phospholipase A and distributed in all the tissues, including hearts [18] . Although previous studies have reported that lysophosphatidylserine has signaling characteristics important in both the early stages of initiating acute inflammation and in the orchestration of its resolution [31] , no previous report has demonstrated its involvement in cell death. Our study shows that lysophosphatidylserine induces necrotic cell death. GPR34 acts as a receptor for lysophosphatidylserine by recognizing its fatty acid at the sn −2 position of the lysophosphatidylserine glycerol backbone [16] . GPR34 is expressed in immune tissues such as lymph nodes, the spleen and thymus, but also in heart tissue [19] . The study presented here showed that GPR34 is activated by lysophosphatidylserine in cardiomyocytes. Previous studies have reported on the functions of GPR34 in inflammatory responses, such as mast cell degranulation [13] and neuro-inflammation [32] . In this study, we show that the knockdown of Gpr34 in isolated cardiomyocytes suppressed lysophosphatidylserine-induced necrosis, but not apoptosis and attenuated lysophosphatidylserine-induced increases in RIP3 and phospho-RIP3 protein levels. Taken together, these results suggest that lysophosphatidylserine induced the activation of G-protein and a signaling pathway towards necrotic cell death in cardiomyocyte. However, it remains to be elucidated the molecular mechanism underlying lysophosphatidylserine-induced and GPR34-mediated necrosis in cardiomyocytes. Furthermore, the ablation of Gpr34 suppressed necrosis in cardiomyocytes and prevented the development of pressure overload-induced cardiomyopathy. These findings indicate that lysophosphatidylserine generated by iPLA 2 β induces necrosis and cardiac dysfunction mediated through the GPR34 signaling pathway. However, it is still unclear whether lysophosphatidylserine induces necrotic cell death in a GPR34-dependent manner in vivo. Although a direct evidence showing causal involvement of lysophosphatidylserine in the phenotype of Pla2g6 −/− mice is required, it is technically difficult to achieve specific reduction of lysophosphatidylserine amount in mouse hearts and to examine the effect of lysophosphatidylserine on cardiac function due to the concomitant induction of severe anaphylaxis reaction, hypothermia and hypotension [14] , [33] . In addition, it remains to be investigated that lysophosphatidylserine might also act as a surfactant or an inflammatory inducer in pressure-overloaded hearts. iPLA 2 β has the important roles in inflammation and other cellular functions/pathologies [34] , [35] , [36] in addition to cell toxicity in cardiomyocytes [21] , [22] , and lysophosphatidylserine generated by iPLA 2 β in fibroblasts or macrophages might act in a paracrine manner on cardiomyocytes. Thus, the role of iPLA 2 β and lysophosphatidylserine in cardiac fibroblasts and/or immune cells using those cell type-specific iPLA 2 β-knockout mice will be investigated in future. In summary, we show that iPLA 2 β plays a detrimental role in the pathogenesis of pressure-overloaded cardiac dysfunction. iPLA 2 β produces 18:0 lysophosphatidylserine, resulting in GPR34-mediated necrotic cell death and cardiac dysfunction. The inhibition of the GPR34 signaling pathway reduces cardiac cell death. Thus, iPLA 2 β, as well as GPR34, may constitute therapeutic targets for patients with heart failure. Study approval All experimental protocols were approved by the Animal Research Committee of Osaka University. All in vivo and in vitro experimental protocols were carried out under the supervision of the Animal Research Committee at Osaka University and in accordance with the Guidelines for Animal Experiments at Osaka University and the Japanese Animal Protection and Management Law. These experiments were performed in accordance with the U.K. Animals (Scientific Procedures) Act 1986 and its associated guidelines, Directive 2010/63/EU for animal experiments. We have complied with ARRIVE (Animal Research: Reporting of In Vivo Experiments) guidelines. Wild-type C57BL/6J (C57BL/6JJmsSlc) mice were purchased from SLC, Japan. All mice were housed in a temperature and humidity-controlled (23 ± 1.5 °C, 45 ± 15%) room with a 12-h light-dark cycle (lights on from 8:00 to 20:00); they were acclimated to the environment at least 7 days before the experiments. Mice were housed in groups with a maximum of five mice per cage and given food (Oriental Yeast, catalog number MF) and water ad libitum . Mice were euthanized in a carbon dioxide-saturated chamber. Generation of cardiomyocyte-specific iPLA 2 β-deficient mice and GPR34-deficient mice The Pla2g6 gene-targeting vector was constructed using C57BL/6J mouse genomic DNA. The targeting construct was developed by inserting the loxP -flippase (FLP) recombinase target (FRT)-neomycin-FRT resistance cassette, a loxP site encompassing exon 10 of the Pla2g6 gene, and the diphtheria toxin A subunit ( DTA ) gene. ES cells (F1; SVJ129 and C57BL/6J) were electroporated with the targeting vector; the transfected ES clones were chosen based on their resistance to diphtheria toxin and neomycin. Circular pCAG-Flpe plasmid was electroporated into the selected ES clones. The screening of the neomycin cassette-excised ES clones was performed by PCR. ES clones exhibiting the desired homologous recombination and normal karyotype were obtained with Southern blotting and karyotyping analyses. To generate chimeric mice, these ES clones were injected into C57BL/6J mouse blastocysts. After the validation of germ line transmission by crossing the chimeric mice with C57BL/6J mice, mice with the floxed Pla2g6 allele were generated. We crossed them with transgenic mice expressing α-myosin heavy chain promoter-driven Cre recombinase ( Myh6-Cre + ) [37] and finally obtained cardiomyocyte-specific iPLA 2 β-deficient mice ( Pla2g6 flox/flox ; Myh6-Cre + , Pla2g6 −/− ). Their Pla2g6 flox/flox ; Myh6-Cre − ( Pla2g6 +/+ ) littermates were used as controls. GPR34-deficient mice [38] were backcrossed to the C57BL/6 background for 12 generations. Only male mice were used in this study. Echocardiography, blood pressure measurement and transverse aortic constriction Echocardiography was performed on conscious mice using an ultrasonographer equipped with a 15-MHz linear transducer (SONOS-4500, Philips Medical Systems). In the two-dimensional parasternal short-axis views, a recording of an M-mode echocardiogram was obtained at the level of the midventricular papillary muscles. To assess left ventricle (LV) size and function, we obtained the following parameters: heart rate (HR), end-diastolic interventricular septum and LV posterior wall thickness (IVSd and LVPWd), end-diastolic and end-systolic LV internal dimensions (LVIDd and LVIDs), and fractional shortening of LV (FS). Blood pressure was non-invasively measured on mice anaesthetized with 2.5% averting using a monitor (MK-2000ST, Muromachi Kikai) according to the manufacturer’s instructions [39] . We performed TAC surgery on male mice aged 10–14 weeks using 27-gauge needles [39] . In brief, anesthesia was induced in mice by administering a combination of ketamine (100 mg/kg) and xylazine (5 mg/kg) intraperitoneally. Mice were then placed under a stereo microscope and intubated for ventilation. Ventilation was provided using a small-animal respirator (model SN-480-7-10; Shinano Seisakusyo) at a rate of 110 cycles per minute, with a tidal volume set at 1 ml per 100 g of body weight. To induce aortic constriction, a 7-0 silk string ligature was tied around a 27-gauge needle, which was subsequently removed. The chest was carefully closed, and the mice were extubated to allow for recovery. Sham-operated animals underwent the same operation without aortic constriction. Careful attention will be paid to healing, analgesia, body weight, surgical wound-sites, hydration, and signs of pain or distress. Isolation of adult cardiomyocytes Using a Langendorff system, adult cardiomyocytes were isolated from male mice at 10 weeks of age [39] . In brief, after anesthesia, the heart was quickly excised from the mice and cannulated via the aorta. Then, the heart was perfused at constant flow for 1 min at 37 °C with a buffer containing 120 mM NaCl (31319, Nakalai Tesque), 5.4 mM KCl (163-03545, FUJIFILM Wako Pure Chemical Corporation), 1.6 mM MgCl 2 (135-00165, FUJIFILM Wako Pure Chemical Corporation), 1.2 mM NaH 2 PO 4 (197-02865, FUJIFILM Wako Pure Chemical Corporation), 5.6 mM glucose (G8270, Sigma-Aldrich), 20 mM NaHCO 3 (191-01305, FUJIFILM Wako Pure Chemical Corporation), and 5 mM taurine (T0625, Sigma-Aldrich), followed by collagenase buffer containing 1.2 mg/ml collagenase type 2 (CLS-2, Worthington Biochemical Corporation) and 0.020 mg/ml protease type XIV (P-5147, Sigma-Aldrich). After filtration into a sterilized tube, the supernatant containing the dispersed myocytes was gently centrifuged at 20 × g for 3 min. The cell pellet was resuspended in the buffer containing 200 μM Ca 2+ . The cardiomyocytes were pelleted by gravity for 10 min. After aspiration of the supernatant, the suspension of rod-shaped cardiomyocytes was then used for western blot analysis or reverse transcription and real-time quantitative polymerase chain reaction (qRT-PCR). Isolation of neonatal rat cardiomyocytes and siRNA transfection We isolated neonatal cardiomyocytes from the ventricles of Kwl/Wistar male rats at 1 day of age (Kiwa Laboratory Animals) [39] . In brief, ventricles were excised from rats and minced with scissors. The cells were dispersed by addition of phosphate-buffered saline containing 0.1% collagenase type 2 and stirred at 37 °C for 10 min. After centrifugation for 5 min, the cells were resuspended in Dulbecco’s modified Eagle’s medium (DMEM) (D5796, Merck Millipore) with 10% fetal bovine serum (FBS) (F7524, Merck Millipore) and filtered through lens papers to remove large clamps of cells. The filtered cells were plated onto culture dishes for 60 min and unattached cells (cardiomyocytes) were removed and replated onto culture dishes. The cells were cultured in DMEM with 10% FBS, 1% penicillin−streptomycin (15140122, Gibco) and 5-Bromo-2’-deoxyuridine (B9285, Sigma-Aldrich). Cultured medium was changed to serum-free medium with penicillin–streptomycin, 5-Bromo-2’-deoxyuridine, transferrin (T3309, Sigma-Aldrich), and insulin (I6634, Sigma-Aldrich) for 48 h after isolation. For knockdown experiments, small-interfering RNA (siRNA) was transfected at 10 nM using transfection reagent (Lipofectamine RNAiMAX transfection reagent, 13778, Invitrogen) 4 h after isolation. siRNAs targeting GPR132, GPR34, and negative control were purchased from Thermo Fisher Scientific (GPR132: catalog number s163527; GPR34: catalog number s181600; negative control: catalog number 4390843). Isolation of primary non-cardiomyocytes Non-cardiomyocytes were isolated from hearts of 10–14-week-old male mice. Ventricles of the hearts were cut into small pieces with scissors followed by digestion using collagenase type 2. The collected cells were suspended in DMEM with 10% FBS and 1% penicillin−streptomycin. The suspended cells were seeded on 6-cm tissue culture dishes. The adherent cells were considered to be non-cardiomyocytes and were used for Western blot analysis [40] . Southern blot analysis Southern blot analysis of embryonic stem cells or mouse hearts was performed [41] . Genomic DNA was purified from embryonic stem cells. Approximately 10 μg of genomic DNA was digested with EcoRI or EcoRV and ran in a 1% agarose gel for 20 h at 30 V. Genomic DNA fragments were transferred from the gel via capillary action to a nylon membrane (0.45 μm pore) using alkaline transfer. The membrane was then exposed to UV light for three minutes for cross-linking. Probes for hybridization were labeled with 32 P-dCTP using the Amersham Megaprime DNA labeling system (GE Healthcare). Hybridization was performed at 68 °C overnight using the QuikHyb Rapid Hybridization solution (Agilent). Western blot analysis Total protein homogenates from the LV, or protein from cells were subjected to western blot analysis. The following antibodies were used in this study: a monoclonal mouse antibody to iPLA 2 β (sc376563, Santa Cruz Biotechnology, Product Clone Name; D-4, 1:100 dilution), a monoclonal mouse antibody to glyceraldehyde-3-phosphate dehydrogenase (GAPDH) (016-25523, FUJIFILM Wako Pure Chemical Corporation, Product Clone Name; 5A12, 1:1000 dilution), a monoclonal mouse antibody to iPLA 2 ζ (MAB3210, Abnova, Product Clone Name; AT2G2, 1:1000 dilution), a polyclonal goat antibody to iPLA 2 ε (EB08402, Everest Biotech, 1:1000 dilution), a polyclonal rabbit antibody to iPLA 2 η (25469-1-AP, Protein Tech, 1:500 dilution), a polyclonal rabbit antibody to iPLA 2 δ (NBP1-74214, Nobus Bio, 1:500 dilution), a polyclonal rabbit antibody to iPLA 2 γ (PA5-49993, Thermo Fisher Scientific, 1:1000 dilution), a polyclonal rabbit antibody to GPR132 (17026-1-AP, Protein Tech, 1:1000 dilution), a polyclonal rabbit antibody to GPR34 (PA5-45717, Thermo Fisher Scientific, 1:1000 dilution), a monoclonal rabbit antibody to RIP1 (#3493, Cell Signaling Technology, Product Clone Name; D94C12, 1:1000 dilution), a polyclonal rabbit antibody to phospho-RIP1 (#31122, Cell Signaling Technology, 1:1000 dilution), a polyclonal rabbit antibody to RIP3 (NBP1-77299, Nobus Bio, 1:1000 dilution), and a monoclonal rabbit antibody to phospho-RIP3 (ab195117, Abcam, Product Clone Name; EPR9516(N)−25, 1:1000 dilution). After incubation with anti-mouse IgG HRP Linked secondary antibody (NA931, Cytiva, 1:10000 dilution) or anti-rabbit IgG HRP Linked secondary antibody (NA934, Cytiva, 1:10000 dilution), the blot was developed with ImmunoStar Zeta or ImmunoStar LD reagent (FUJIFILM Wako Pure Chemical Corporation) and observed using ImageQuant LAS4000mini (Cytiva). The expression levels of protein were evaluated using ImageQuantTL (version 7.0, Cytiva). Uncropped and unprocessed scans of blots are supplied in the Source Data file or as a supplementary figure in the Supplementary Information. Histological analysis The heart tissues were fixed in 10% neutral buffered formalin. The samples were embedded in paraffin and cut into 5-μm sections. Serial sections were stained with hematoxylin and eosin, wheat germ agglutinin (W11261, Thermo Fisher Scientific), or Azan-Mallory staining [42] . Quantitation of the cardiomyocyte cross-sectional area was conducted by tracing the outline of 200—250 myocytes in each section, while quantitative analysis of fibrosis was performed in the whole area of sections using ImageJ (version 1.51j8, National Institutes of Health) [42] . The TUNEL assay was performed using the In Situ Cell Death Detection Kit, Fluorescein (11684795910, Roche) with a mouse monoclonal antibody to α-sarcomeric actin (A2172, Thermo Fisher Scientific, Product Clone Name; 5C5, 1:500 dilution) and anti-mouse IgM Texas Red® conjugated antibody (Tl2020, Vector Laboratory, 1:10 dilution); the sections were mounted with VECTASHIELD with DAPI (H-1200, Vector Laboratories). These samples were observed under an FV-1000D microscope (Olympus); the numbers of TUNEL–positive nuclei and total nuclei were counted. For immunohistochemical analysis of inflammatory cell infiltration into the heart, frozen heart sections (5 μm thickness) were fixed in buffered 4% paraformaldehyde. We used primary antibodies—anti-mouse CD45 (103101, Biolegend, Product Clone Name; 30-F11, 1:100 dilution), CD68 (MCT1957T, Bio-Rad, Product Clone Name; FA-11, 1:100 dilution), Ly6G/6C (550291, BD Pharmingen, Product Clone Name; RB6-8C5, 1:100 dilution), CD3 (ab16669, Abcam, Product Clone Name; SP7, 1:100 dilution)—and secondary antibodies—anti-rat IgG or anti-rabbit IgG biotinylated antibodies (BA-4001 or BA-1000, Vector Laboratory, 1:200 dilution)—along with avidin-peroxidase (Vectastain Elite ABC Kit, Vector Laboratories) and ImmPACT DAB Peroxidase Substrate Kit (SK-4105, Vector Laboratories), followed by counterstaining with Meyer’s Hematoxylin solution (MHS-1, Sigma-Aldrich) and mounting with Entellan (107960, Merck Millipore). Microscopic analysis was performed using BZX710 or 810 (Keyence) [39] . Quantitative analyses of inflammatory cells were examined by counting the number of immunopositive cells in an entire section. For immunohistochemical analysis of necrosis, frozen heart sections (5 μm thickness) were fixed in buffered 4% paraformaldehyde. The primary and secondary antibody used was a polyclonal rabbit antibody to HMGB1 (ab18256, Abcam, 1:100 dilution) and anti-rabbit IgG Alexa Fluor™ 488 conjugated antibody (A11034, Invitrogen, 1:100 dilution). Heart sections were also reacted with a mouse monoclonal antibody to α-sarcomeric actin and were then mounted with VECTASHIELD with DAPI. These sections were observed under an FV-1000D microscope. For Evans blue staining, mice were injected intraperitoneally with Evans blue dye (1 mg/0.1 ml PBS/10 g body weight, 056-04061, FUJIFILM Wako Pure Chemical Corporation) 24 h before sacrifice. Serial frozen sections (5 μm thickness) of the hearts were fixed in buffered 4% paraformaldehyde and mounted with VECTASHIELD with DAPI. These sections were observed under BZX710 and analyzed for dye uptake using Image J. Serum cardiac troponin T Blood samples were obtained from the inferior venae cava of mice using non-heparinized syringes. The blood samples were left for 1 h at room temperature and stored at 4 °C overnight. Serum was collected after centrifuging at 1200 × g for 30 min. Serum cardiac troponin T was measured at the SRL, Inc (Tokyo, Japan) Reverse transcription and real-time quantitative polymerase chain reaction (qRT-PCR) Total RNA was isolated from the LV tissue or cardiomyocytes using TRIzol reagent (15596026, Thermo Fisher Scientific). To remove residual reagent and DNA, we used DNase (313-03161, Nippon Gene) and a nuclear clean up kit (740948, Macherey-Nagel). The amounts of acquired total RNA were measured via Nanodrop 1000 spectrophotometer (Thermo Fisher Scientific). 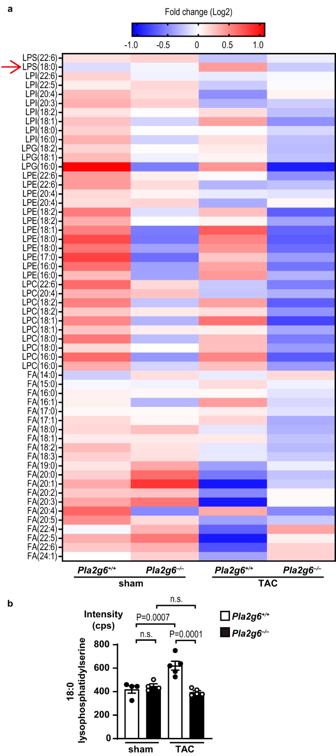Fig. 4: Untargeted lipidomic analysis of free fatty acids and lysophospholipids released in TAC-operatedPla2g6−/−heart tissue. aHeat map showing the contents of molecular species of free fatty acids and lysophospholipids in mouse hearts after TAC operation. Correlation of peak values and color is indicated at the top; High, red and low, blue. Red arrow indicates 18:0 lysophosphatidylserine. LPS lysophosphatidylserine, LPI lysophosphatidylinositol, LPG lysophosphatidylglucoside, LPE lysophosphatidylethanolamine, LPC lysophosphatidylcholine, FA free fatty acid.bQuantity of 18:0 lysophosphatidylserine in mouse hearts after TAC operation.n= 4 (sham-operatedPla2g6+/+), 4 (sham-operatedPla2g6–/–), 5 (TAC-operatedPla2g6+/+), and 5 (TAC-operatedPla2g6–/–), biologically independent samples. Average values of each group were used for heat map analysis (a). Open and closed bars indicatePla2g6+/+andPla2g6−/−, respectively (b). Data are expressed as the mean ± SEM. The data were evaluated by one-way ANOVA, followed by Tukey-Kramer’spost-hoctest. Source data are provided as a Source Data file. The mRNA expression levels were determined via reverse transcription polymerase chain reaction (PCR) using MultiScribe Reverse Transcriptase (4374966, Applied Biosystems) and via quantitative PCR using the Power-Up SYBR Green Master Mix (a25742, Applied Bio Systems) [43] ; the PCR primers used are shown in the primer list (Supplementary Table 4 ). The mRNA expression levels were measured using QuantStudio 7 Flex (Applied Biosystems) and were calculated in QuantStudio Realtime PCR software (Applied Bio Systems). All data were normalized to the Gapdh mRNA expression level and are expressed as the fold increase over the control group. Lipidomic analysis Untargeted lipidomics was performed using a single-phase lipid extraction method [44] . In brief, 200 μl of suspension from each heart tissue in methanol containing internal standards was mixed with 100 μl chloroform and incubated for 1 h at room temperature. Subsequently, 20 μl of water was added, before the samples were incubated for 10 min and then centrifuged at 2000 × g for 10 min. The supernatants were collected and analyzed using an ACQUITY UPLC system (Waters, Milford, MA) coupled with a QTOF-MS (TripleTOF 6600; Sciex, Framingham, MA). The flow rate was 300 μl/minute at 45 °C, while the injection volume was 2 μl. The information-dependent acquisition (IDA) mode was applied to confirm each of the lipid profiles and structures in negative-ion mode. Targeted lipidomics for PUFA metabolites were performed using an ACQUITY UPLC system (Waters) with a linear ion-trap quadrupole mass spectrometer (QTRAP5500; Sciex) [45] . Samples were prepared by solid-phase extraction with a Sep-Pak C18 cartridge (Waters) using deuterium-labeled internal standards. MS/MS analyses were conducted in negative-ion mode. Fatty acid metabolites were identified and quantified by multiple reaction monitoring (MRM). Data were collected and analyzed using Analyst TF v1.8.1 and Analyst Software v1.6 (SCIEX) and MultiQuant software v2.0 (SCIEX), SCIEX MS data converter v1.3 beta (SCIEX), and 2DICAL v0.91 (Mitsui Knowledge Industry), respectively. Additional details regarding the lipidomics analysis are provided in the checklist of the supplementary information file. Cell viability assay Rat neonatal cardiomyocytes were stimulated with 18:0 lysophosphatidylserine (858144 P, Avanti Polar Lipid). After designated periods or concentrations of drug exposure, Cell Titer Blue reagent (G8081, Promega) was added into culture medium 90 min before measurement. Cell viabilities were estimated by measuring the intensity of fluorescence (excitation 560 nm, emission 590 nm) using a microplate reader (SH-9000lab, Hitachi High-Tech Science Corporation). In vitro immunofluorescence microscopy Neonatal rat cardiomyocytes were cultured on glass-based dishes (3910-035, IWAKI Cell Biology) and incubated with 50 μM 18:0 lysophosphatidylserine. To visualize apoptosis and necrosis, the cells were incubated in 3D gel with Cell-matrix I-A (KURABO INDUSTRIES) and stained with propidium iodide (341-07881, FUJIFILM Wako Pure Chemical Corporation) for 5 min before fixation with methanol at −30 °C for 15 min. The cells were stained using TUNEL before confocal microscopic analysis using an FV-1000D microscope [39] . Cyclic-AMP assay Neonatal rat cardiomyocytes were seeded onto six-well plates. Cells were stimulated with 10 μM forskolin (067-02191, FUJIFILM Wako Pure Chemical Corporation) for 20 min before treatment with indicated concentrations of 18:0 lysophosphatidylserine for 10 min at 37 °C. The accumulated cAMP concentrations were measured using a cAMP assay kit (Abcam ab290713) according to the manufacturer’s instruction. Statistical analysis Data are shown as the mean ± SEM. GraphPad Prism (version 8.4.3, GraphPad Software, La Jolla, California) was used for statistical analysis. The Kaplan-Meier method with the log-rank test was used for survival analysis. Two-sided unpaired Student’s t- test was used for 2-group comparison. We used one-way analysis of variance (ANOVA) followed by Tukey-Kramer’s post - hoc test or two-way ANOVA followed by Bonferroni’s post - hoc test for multiple comparisons. 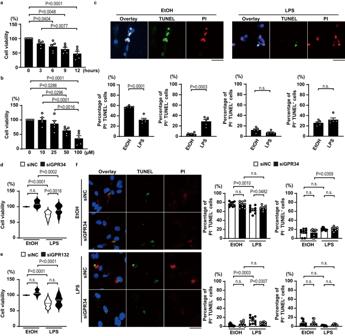Fig. 5: 18:0 lysophosphatidylserine-induced cell death in rat neonatal cardiomyocytes. a,bCell viability assay. Cell viability was measured using the Cell Titer-Blue Assay Kit. Isolated rat neonatal cardiomyocytes were treated with 50 μM 18:0 lysophosphatidylserine for the indicated time, or with the indicated concentration of 18:0 lysophosphatidylserine for 12 h. The percentage of cell viability is shown in the graphs (n= 5). The data were evaluated by one-way ANOVA, followed by Tukey-Kramer’spost-hoctest.cImmunofluorescent analysis of TUNEL (green), propidium iodide (PI) (red) and DAPI (blue) stained-neonatal cardiomyocytes after stimulation with 50 μM 18:0 lysophosphatidylserine (LPS) for 12 h. Scale bars, 50 μm. Necrosis was assessed by PI+and TUNEL–, while early apoptosis was assessed by PI–and TUNEL+and late apoptosis was assessed by PI+and TUNEL+. The bottom graphs show quantitative analysis (n= 5). Two-sided unpaired Student’st-test was used for analysis (EtOH versus LPS in Percentage of PI–TUNEL–cellsP= 0.00006). 1% (v/v) ethanol (EtOH) was used as the control sample.d,eThe effect of knockdown of LPS receptors on cell viability. Isolated neonatal cardiomyocytes were transfected with siRNAs targeting GPR34 or GPR132 (siGPR34 or siGPR132) or with negative control siRNA (siNC). These cells were treated with 50 μM LPS for 12 h. The percentage of cell viability is shown in the graphs (n= 12). The data were analyzed by one-way ANOVA, followed by Tukey-Kramer’spost-hoctest (siNC EtOH versus siNC LPS in (d,e)P= 0.0000005 andP= 0.0000007, respectively, siGPR132 EtOH versus siGPR132 LPSP= 0.000002). Open and closed bars indicate siNC and siGPR34 or siGPR132, respectively.fImmunofluorescent analysis of TUNEL, PI and DAPI stained-cardiomyocytes after stimulation with 50 μM LPS for 12 h under the condition of GPR34 knockdown. Scale bar, 50 μm. The graphs show quantitative analysis (n= 9). The data were evaluated by one-way ANOVA, followed by Tukey-Kramer’spost-hoctest. Open and closed bars indicate siNC and siGPR34, respectively. In violin plots, solid lines show median. In bar graphs, data are expressed as the mean ± SEM. Source data are provided as a Source Data file. 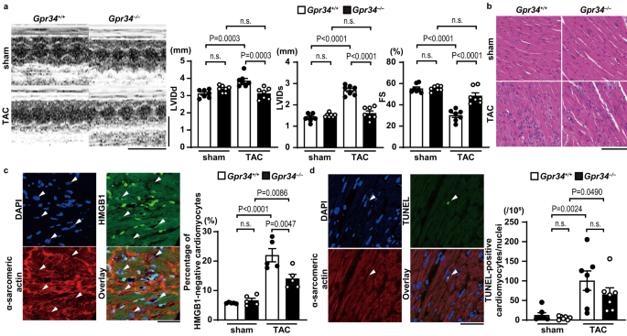Fig. 6: The protective effect of GPR34 deficiency from pressure overload in the heart. Gpr34+/+andGpr34–/–mice were subjected to TAC and then analyzed 5 days after the operation.aRepresentative images of transthoracic M-mode echocardiographic tracing. Scale bars, 0.2 s and 5 mm, respectively. The graphs show echocardiographic parameters of the mice (n= 7, biologically independent samples. ShamGpr34+/+versus TACGpr34+/+in LVIDs and FSP= 0.0000000001 andP= 0.0000002, respectively, TACGpr34+/+versus TACGpr34–/–in LVIDs and FSP= 0.000000006 andP= 0.00006, respectively).bRepresentative images of the hematoxylin-eosin-stained heart sections. Experiment was repeated five times independently with similar results. Scale bar, 100 μm.cImmunofluorescence analysis of HMGB1 (green), α-sarcomeric actin (red) and DAPI (blue) in the heart after TAC (n= 5, biologically independent samples. ShamGpr34+/+versus TACGpr34+/+P= 0.000002). Arrow heads indicate HMGB1-negative nuclei. Scale bar, 50 μm. The graph shows the percentage of HMGB1-negative cardiomyocytes.dRepresentative confocal images of TUNEL (green)-positive cardiomyocytes. Arrow heads indicate TUNEL-positive nuclei. Scale bar, 50 μm. Red, α-sarcomeric actin; blue, DAPI. The graph shows quantitative analysis of TUNEL-positive cardiomyocytes. (n= 7, biologically independent samples). Open and closed bars indicateGpr34+/+andGpr34−/−, respectively. Data are expressed as the mean ± SEM. The data were evaluated by one-way ANOVA, followed by Tukey-Kramer’spost-hoctest. Source data are provided as a Source Data file. P < 0.05 was considered statistically significant. Reporting summary Further information on research design is available in the Nature Portfolio Reporting Summary linked to this article.